Lysophospholipids secreted by splenic macrophages induce chemotherapy resistance via interference with the DNA damage response Host responses to systemic anti-cancer treatment play important roles in the development of anti-cancer drug resistance. Here we show that F4/80 + /CD11b low splenocytes mediate the resistance to DNA-damaging chemotherapeutics induced by two platinum-induced fatty acids (PIFAs), 12-S-keto-5,8,10-heptadecatrienoic acid and 4,7,10,13-hexadecatetraenoic acid (16:4(n−3)) in xenograft mouse models. Splenectomy or depletion of splenic macrophages by liposomal clodronate protects against PIFA-induced chemoresistance. In addition, we find that 12-S-HHT, but not 16:4(n−3), functions via leukotriene B4 receptor 2 (BLT2). Genetic loss or chemical inhibition of BLT2 prevents 12-S-HHT-mediated resistance. Mass spectrometry analysis of conditioned medium derived from PIFA-stimulated splenic macrophages identifies several lysophosphatidylcholines as the resistance-inducing molecules. When comparing cisplatin and PIFA-treated tumours with cisplatin alone treated tumours we found overall less γH2AX, a measure for DNA damage. Taken together, we have identified an intricate network of lysophospholipid signalling by splenic macrophages that induces systemic chemoresistance in vivo via an altered DNA damage response. The development of resistance to chemotherapy is one of the most important obstacles to continued effective treatment of cancer in patients. Resistance to treatment is generally considered to be the result of tumour-intrinsic alterations in which tumour cells acquire genetic mutations, leading to treatment tolerance or utilization of compensatory pathways to become drug tolerant. During recent years, it has become clear that in addition to tumour cell intrinsic resistance, signalling events from the tumour microenvironment play a major role in drug resistance [1] , [2] , [3] , [4] . Macrophages are highly plastic cells that adopt a tumour promoting or tumour-inhibiting phenotype, depending on the surrounding stimuli [5] . Macrophages can infiltrate developing tumours in large numbers and these tumour-associated macrophages (TAMs) can hamper chemotherapy via various mechanisms involving cathepsins, colony stimulating factor 1 (CSF1) and metalloproteases [6] , [7] , [8] , [9] . Recently, Cortez-Retamozo et al. [10] showed that the spleen harbours TAM precursors which play an important role in tumour progression. Furthermore, Ugel et al. [11] have shown that CD11b + /GR1 int /Ly6C high cells residing in the marginal zone of the spleen play a key role in generating tolerance to tumour antigens and that splenectomy prevents tumour-induced tolerance. In general, TAMs are considered to exert their effects locally. In this study we show that macrophages residing in the spleen can be specifically activated by circulating fatty acids to secrete secondary lysophospholipids which lead to systemic resistance to genotoxic chemotherapy. PIFAs protect only against DNA-damaging chemotherapeutics We have found that mesenchymal stem cells (MSCs) can secrete two specific polyunsaturated fatty acids in response to platinum-containing chemotherapeutics and that these platinum-induced fatty acids (PIFAs) can independently induce resistance to various chemotherapeutics at minute quantities ( Supplementary Fig. 1 and Roodhart et al. [12] ). To determine whether the effects of PIFAs are limited to DNA-damaging agents, we tested two non-genotoxic agents, paclitaxel (spindle poison) and sorafenib (tyrosine kinase inhibitor), and found that their anti-tumour effects were not inhibited by co-administration of PIFAs ( Fig. 1a,b ). This suggested that PIFAs specifically protect against the effects of DNA-damaging agents. To further investigate this effect we analyzed γH2AX foci, which mark DNA damage. Treatment with cisplatin resulted in a strong increase in the number of γH2AX-positive cells over time with a peak at 4 h after treatment. Co-treatment with PIFAs largely reversed the cisplatin-induced DNA damage ( Fig. 1c ). In line with these findings BrdU and phospho-histone 3 (pH3) levels were higher in tumours treated with cisplatin and PIFAs compared with tumours treated with cisplatin alone ( Supplementary Fig. 2 ). Flow cytometric analyses of single cell suspensions of mouse tumours showed that 8 h after therapy, in cisplatin-treated tumours high percentages of cells were in subG1 or in a G1/S arrest, whereas in tumours treated with cisplatin and PIFAs, cell cycle profiles were comparable to the untreated controls ( Fig. 1d ). The difference in γH2AX was not the result of an altered exposure to cisplatin. Cytosolic, nuclear and DNA-bound platinum concentrations were similar in presence or absence of PIFAs 1 h after treatment ( Fig. 1e ). Previously published data showed that PIFAs exert their effects even when administered up to 4 h after cisplatin treatment [12] . 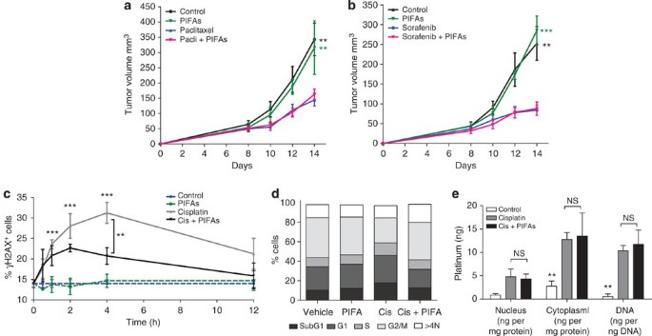Figure 1: PIFAs induce chemoresistance by interfering with the DNA damage response. Co-administration of PIFAs with non-DNA-damaging agents paclitaxel (a) or sorafenib (b) did not induce chemoresistance. Immunohistochemical analysis of tumours stained for γH2AX showed decrease in γH2AX over time after co-treatment with cisplatin and PIFAs compared with cisplatin treatment (c). Single cell suspensions were prepared from tumours and stained with propidium iodide for flow cytometric analysis of cell cycle profiles. Cisplatin-treated tumours are arrested in subG1 and G1/S phase, whereas the tumours receiving a combination of cisplatin and PIFAs show cell cycle profiles comparable to control animals (d). Platinum concentration in the cytoplasm, nucleus or bound to DNA was determined by inductively coupled plasma mass spectrometry, revealing no differences between cisplatin alone treatment and cisplatin+PIFAs (e). All graphs show results of two independent experiments (n=8 per group). All experiments were performed in C26 tumour-bearing balb/c mice. Data are represented as mean±s.e.m. Statistical significance was determined by one-way analysis of variance or two-tailed Studentst-test. All cisplatin alone unless indicated otherwise *P<0.05, **P<0.01, ***P<0.001. Figure 1: PIFAs induce chemoresistance by interfering with the DNA damage response. Co-administration of PIFAs with non-DNA-damaging agents paclitaxel ( a ) or sorafenib ( b ) did not induce chemoresistance. Immunohistochemical analysis of tumours stained for γH2AX showed decrease in γH2AX over time after co-treatment with cisplatin and PIFAs compared with cisplatin treatment ( c ). Single cell suspensions were prepared from tumours and stained with propidium iodide for flow cytometric analysis of cell cycle profiles. Cisplatin-treated tumours are arrested in subG1 and G1/S phase, whereas the tumours receiving a combination of cisplatin and PIFAs show cell cycle profiles comparable to control animals ( d ). Platinum concentration in the cytoplasm, nucleus or bound to DNA was determined by inductively coupled plasma mass spectrometry, revealing no differences between cisplatin alone treatment and cisplatin+PIFAs ( e ). All graphs show results of two independent experiments ( n =8 per group). All experiments were performed in C26 tumour-bearing balb/c mice. Data are represented as mean±s.e.m. Statistical significance was determined by one-way analysis of variance or two-tailed Students t -test. All cisplatin alone unless indicated otherwise * P <0.05, ** P <0.01, *** P <0.001. Full size image The spleen is involved in PIFA-mediated chemoresistance In search for a mechanism we noted that the PIFAs failed to induce chemoresistance in an experimental liver metastasis model using the same tumour cells and mouse strain as our subcutaneous model in which resistance is seen ( Fig. 2a,b ). In this metastasis model tumour cells are injected in the spleen to allow venous access to the liver, after which the spleen is removed to avoid local tumour growth. This observation combined with our findings that PIFAs could not cause resistance directly to tumour cells in vitro ( Fig. 2c ) suggested an indirect mechanism involving the spleen. Indeed, 16:4(n−3) and 12-S-HHT failed to induce resistance to chemotherapy in splenectomized, tumour-bearing mice ( Fig. 2d ). To re-introduce chemoresistance we treated splenectomized tumour-bearing mice with chemotherapy alone or in combination with conditioned medium obtained from full spleen cell suspensions incubated in the presence (sCM + ) or absence (sCM − ) of both PIFAs. sCM + from full spleen was able to induce chemoresistance in vivo in splenectomized mice, whereas sCM − was not ( Fig. 2e ). In addition, we found that sCM + from human splenocytes incubated with both PIFAs could also induce chemoresistance in splenectomized mice, indicating potential clinical translation ( Fig. 2f ). 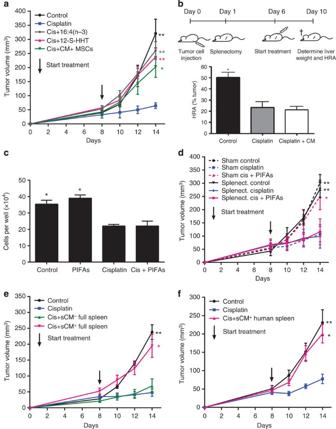Figure 2: The spleen is required for PIFA-induced chemoresistance. 12-S-HHT and 16:4(n−3) induce chemoresistance individuallyin vivoin C26 tumour-bearing balb/c mice. CM+derived from MSCs stimulated with cisplatin also induces chemoresistancein vivo(a). CM+from MSCs does not cause resistance in liver metastasis model in which the spleen is removed (b). PIFAs cannot induce resistance directly on C26 tumour cellsin vitro(c). Cells were plated in 24-well plate on the day prior to cisplatin and/or PIFAs treatment. Twenty-four hours after treatment with cisplatin (3 μM) alone or in combination with PIFAs (HHT 20 nM, 16:4(n−3) 25 nM) the cells were harvested and counted. Splenectomy protects against PIFA-mediated chemoresistance in C26 tumour-bearing balb/c mice (d). sCM+from full spleen can restore resistance in splenectomized tumour-bearing mice, whereas sCM−cannot (e). sCM+from human splenocytes induces resistance in splenectomized mice (f). For all experiments C26 tumour-bearing balb/c mice were used.a,c–eshow results of three independent experiments with similar outcome (n=12 per group).b,fshow results from two independent experiments with similar outcome (n=8 per group forb,n=9 per group forf). Data are represented as mean±s.e.m. Statistical significance was determined by one-way analysis of variance. All compared with cisplatin alone, *P<0.05, **P<0.01. Figure 2: The spleen is required for PIFA-induced chemoresistance. 12-S-HHT and 16:4(n−3) induce chemoresistance individually in vivo in C26 tumour-bearing balb/c mice. CM + derived from MSCs stimulated with cisplatin also induces chemoresistance in vivo ( a ). CM + from MSCs does not cause resistance in liver metastasis model in which the spleen is removed ( b ). PIFAs cannot induce resistance directly on C26 tumour cells in vitro ( c ). Cells were plated in 24-well plate on the day prior to cisplatin and/or PIFAs treatment. Twenty-four hours after treatment with cisplatin (3 μM) alone or in combination with PIFAs (HHT 20 nM, 16:4(n−3) 25 nM) the cells were harvested and counted. Splenectomy protects against PIFA-mediated chemoresistance in C26 tumour-bearing balb/c mice ( d ). sCM + from full spleen can restore resistance in splenectomized tumour-bearing mice, whereas sCM − cannot ( e ). sCM + from human splenocytes induces resistance in splenectomized mice ( f ). For all experiments C26 tumour-bearing balb/c mice were used. a , c – e show results of three independent experiments with similar outcome ( n =12 per group). b , f show results from two independent experiments with similar outcome ( n =8 per group for b , n =9 per group for f ). Data are represented as mean±s.e.m. Statistical significance was determined by one-way analysis of variance. All compared with cisplatin alone, * P <0.05, ** P <0.01. Full size image Spleen macrophages are required for PIFA-mediated resistance in vivo Next, we tested individual splenic cell populations for their potential to induce resistance in vivo . We tested natural killer cells (CD49 + cells), dendritic cells (CD11c + cells), macrophages (F4/80 + cells), monocytes (CD11b + cells), metallophilic marginal zone macrophages (CD169 + cells) and T and B cells (CD3 + and B220 + cells). Only the sCM + of F4/80 + splenocytes was able to significantly induce resistance in vivo ( Fig. 3a ). Furthermore, none of the sCM − samples were able to induce resistance in vivo ( Fig. 3b ). Importantly, treatment with either PIFAs or sCM alone did not alter tumour growth ( Fig. 3c ). Further refinement of the F4/80 + cell population by fluorescence-activated cell sorting (FACS) indicated a role for F4/80 + /CD11b low macrophages ( Fig. 3d ). In addition, we used liposomal clodronate to deplete F4/80 + /CD11b low splenocytes. Depletion of F4/80 + /CD11b low splenocytes had no direct effect on tumour growth in vitro and in vivo ( Supplementary Fig. 3 ), but potently reversed the PIFA-induced chemoresistance to cisplatin in both C26 tumour-bearing balb/c mice and LLC tumour-bearing C57bl/6 mice ( Fig. 3e,f ). Chemoresistance was re-instated when liposomal clodronate-treated mice were injected with sCM + from PIFA-stimulated F4/80 + splenocytes ( Fig. 3e,f ). 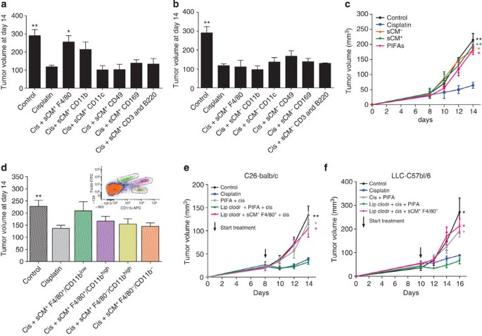Figure 3: Splenic F/80+/CD11blowmacrophages play a key role in chemoresistance induced by PIFAs. sCM+from F4/80+splenocytes significantly restored resistance in splenectomized tumour-bearing mice, whereas sCM+from other splenic populations cannot (a). sCM−from any of the isolated populations is unable to induce resistance (b). In addition, PIFAs, sCM−or sCM+alone do not affect normal tumour growth (c). sCM+from FACS-sorted F4/80+/CD11blow, F4/80+/CD11bhigh, F4/80−/CD11bhighand F4/80−/CD11b−splenocytes did not significantly induce chemoresistance, however F4/80+/CD11blowcells were most potent (d, insert shows gated populations). Animals treated with liposomal clodronate and cisplatin+PIFAs remained chemosensitive. sCM+from F4/80+cells rescued loss of resistance in liposomal clodronate-treated mice (cis+sCM+F4/80+).eshows results from C26-balb/c model andfshows results from LLC-C57bl/6 model. All graphs show data from C26-balb/c model unless indicated otherwise. Graphs ina,d–fshow results of three independent experiments with similar outcome (n=12 per group). Graphs inb,cshow results of two independent experiments with similar outcome (n=10 per group). Data are represented as mean±s.e.m. Statistical significance was determined by one-way analysis of variance. All compared with cisplatin alone, *P<0.05, **P<0.01. Figure 3: Splenic F/80 + /CD11b low macrophages play a key role in chemoresistance induced by PIFAs. sCM + from F4/80 + splenocytes significantly restored resistance in splenectomized tumour-bearing mice, whereas sCM + from other splenic populations cannot ( a ). sCM − from any of the isolated populations is unable to induce resistance ( b ). In addition, PIFAs, sCM − or sCM + alone do not affect normal tumour growth ( c ). sCM + from FACS-sorted F4/80 + /CD11b low , F4/80 + /CD11b high , F4/80 − /CD11b high and F4/80 − /CD11b − splenocytes did not significantly induce chemoresistance, however F4/80 + /CD11b low cells were most potent ( d , insert shows gated populations). Animals treated with liposomal clodronate and cisplatin+PIFAs remained chemosensitive. sCM + from F4/80 + cells rescued loss of resistance in liposomal clodronate-treated mice (cis+sCM + F4/80 + ). e shows results from C26-balb/c model and f shows results from LLC-C57bl/6 model. All graphs show data from C26-balb/c model unless indicated otherwise. Graphs in a , d – f show results of three independent experiments with similar outcome ( n =12 per group). Graphs in b , c show results of two independent experiments with similar outcome ( n =10 per group). Data are represented as mean±s.e.m. Statistical significance was determined by one-way analysis of variance. All compared with cisplatin alone, * P <0.05, ** P <0.01. Full size image Further characterization of the F4/80 + /CD11b low splenocytes showed that they are localized in the red pulp and lack Ly6G and Ly6C expression ( Supplementary Fig. 4 ). Analysis of the number of F4/80 + infiltrating cells in both our subcutaneous tumours showed very little infiltrating macrophages in both LLC and C26 tumours ( Supplementary Fig. 5 ), suggesting that in our xenograft models the contribution of TAMs is unlikely. We thus conclude that 12-S-HHT and 16:4(n−3) signal via macrophages residing in the spleen to confer chemoresistance. Loss of BLT2 blocks 12-S-HHT-mediated chemoresistance Leukotriene B4 receptor 2 (BLT2) is the low affinity receptor for leukotriene B4, but also specifically binds 12-S-HHT and initiates distinct events, setting it apart from BLT1 (ref. 13 ). Given the fact that 12-S-HHT is a natural ligand of BLT2 (ref. 14 ) we focused on the interaction between BLT2 and 12-S-HHT in splenic macrophage-induced resistance. Analysis of expression levels showed that BLT2 is exclusively expressed on F4/80 + /CD11b low splenocytes ( Fig. 4a ). sCM + from splenic macrophages cultured in the presence of LY255283, a BLT2 antagonist, and 12-S-HHT failed to induce resistance in splenectomized mice. In contrast, sCM + from spleen macrophages cultured in the presence of BLT1 antagonist U-75302 and 12-S-HHT retained resistance-inducing potential ( Fig. 4b ). Importantly, 16:4(n−3)-mediated resistance was not hampered by the two antagonists ( Fig. 4c ). To further confirm the interaction between 12-S-HHT and BLT2 we tested the PIFAs in BLT2 −/− mice. We found that 12-S-HHT-mediated resistance was lost in BLT2 −/− LLC tumour-bearing mice, whereas 16:4(n−3) fully retained its ability to induce resistance ( Fig. 4d ). We also showed that sCM + from BLT2 −/− splenocytes incubated with 12-S-HHT was unable to cause resistance in wild-type C57bl/6 mice, whereas the resistance-inducing potential of sCM + from BLT2 −/− spleens incubated with 16:4(n−3) was unaffected ( Supplementary Fig. 4e ). Noteworthy, the tumour growth was delayed in BLT2 −/− mice compared with wild-type mice ( Supplementary Fig. 6 ). As expected, 12-S-HHT and 16:4(n−3) could reduce γH2AX levels in cisplatin-treated tumours in the parental C57bl/6 strain ( Fig. 5a ). Interestingly, tumours in BLT2 −/− mice that received cisplatin and 12-S-HHT had comparable γH2AX levels to mice treated with cisplatin alone, whereas 16:4(n−3) and cisplatin-treated tumours showed decreased γH2AX levels ( Fig. 5b ). This further emphasizes that BLT2 signalling is essential in facilitating 12-S-HHT-mediated chemoresistance via alteration of the DNA damage response. 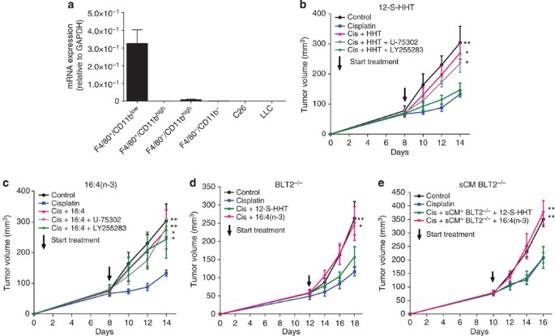Figure 4: Inhibition or loss of BLT2 blocks formation of 12-S-HHT-induced resistance. BLT2 is exclusively expressed on F4/80+/CD11blowsplenocytes as was shown by quantitative PCR (a). Incubation of splenocytes with LY255283 and 12-S-HHT blocked 12-S-HHT-induced resistance, whereas U-75302 did not (b). Neither U-75302 nor LY255283 blocked 16:4(n−3)-mediated chemoresistance (c). 12-S-HHT failed to induce resistance in BLT2−/−mice (d). Co-administration of cisplatin with sCM+from BLT2−/−mice incubated with 12-S-HHT did not induce resistance in wild-type C57bl/6 mice, whereas sCM+from BLT2−/−incubated with 16:4(n−3) does induce chemoresistance (e). Graphs depicted show data from two independent experiments (a,n=4 per group,b–e,n=10 per group). Statistical significance was determined by one-way analysis of variance or two-tailed Studentst-test. All compared with cisplatin alone. *P<0.05, **P<0.01. Figure 4: Inhibition or loss of BLT2 blocks formation of 12-S-HHT-induced resistance. BLT2 is exclusively expressed on F4/80 + /CD11b low splenocytes as was shown by quantitative PCR ( a ). Incubation of splenocytes with LY255283 and 12-S-HHT blocked 12-S-HHT-induced resistance, whereas U-75302 did not ( b ). Neither U-75302 nor LY255283 blocked 16:4(n−3)-mediated chemoresistance ( c ). 12-S-HHT failed to induce resistance in BLT2 −/− mice ( d ). Co-administration of cisplatin with sCM + from BLT2 −/− mice incubated with 12-S-HHT did not induce resistance in wild-type C57bl/6 mice, whereas sCM + from BLT2 −/− incubated with 16:4(n−3) does induce chemoresistance ( e ). Graphs depicted show data from two independent experiments ( a , n =4 per group, b – e , n =10 per group). Statistical significance was determined by one-way analysis of variance or two-tailed Students t -test. All compared with cisplatin alone. * P <0.05, ** P <0.01. 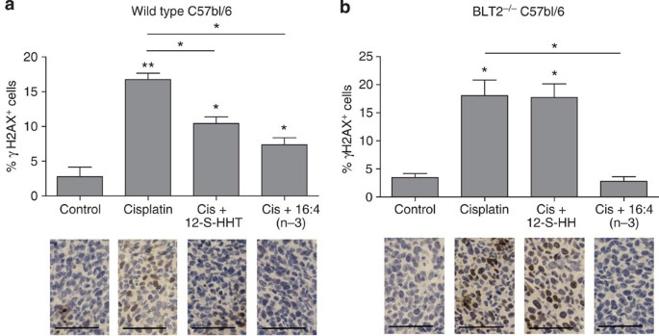Figure 5: BLT2−/−mice are unresponsive to 12-S-HHT mediated alterations in DNA damage response. Co-treatment of wild-type mice with 12-S-HHT or 16:4(n−3) and cisplatin decreased γH2AX levels compared with cisplatin (a). In BLT2−/−mice γH2AX levels were comparable between 12-S-HHT and cisplatin co-treatment and cisplatin treatment (b). Mice were killed 4 h after treatment with cisplatin and/or 12-S-HHT or 16:4(n−3). Tumours were stained for γH2AX and quantified. Graphs depicted show data from two independent experiments (n=4 per group). Scale bars, 50 μm. Statistical significance was determined by two-tailed Studentst-test. All compared with cisplatin alone unless indicated otherwise. *P<0.05, **P<0.01. Full size image Figure 5: BLT2 −/− mice are unresponsive to 12-S-HHT mediated alterations in DNA damage response. Co-treatment of wild-type mice with 12-S-HHT or 16:4(n−3) and cisplatin decreased γH2AX levels compared with cisplatin ( a ). In BLT2 −/− mice γH2AX levels were comparable between 12-S-HHT and cisplatin co-treatment and cisplatin treatment ( b ). Mice were killed 4 h after treatment with cisplatin and/or 12-S-HHT or 16:4(n−3). Tumours were stained for γH2AX and quantified. Graphs depicted show data from two independent experiments ( n =4 per group). Scale bars, 50 μm. Statistical significance was determined by two-tailed Students t -test. All compared with cisplatin alone unless indicated otherwise. * P <0.05, ** P <0.01. Full size image Splenic chemoresistance factors are lysophosphatidylcholines To identify the secondary molecules secreted by PIFA-stimulated splenic macrophages we applied a stepwise fractionation of the sCM + ( Fig. 6a ). We found that the total lipid fraction, but not the protein-containing fraction, extracted from sCM + induced resistance in splenectomized mice, whereas the total lipid fraction from sCM − did not. In line with these results we found that delipidation of sCM + resulted in a loss of chemoresistance-inducing potential ( Fig. 6b ), indicating that the secondary molecules are lipids. A solid phase-based fractionation of the total lipid fraction into neutral lipids, free fatty acids and two phospholipid fractions (phosphatidylcholines, phoshatidylethanolamines and sphingomyelines (PC/PE/SM) and phosphatidylinositol, phosphatidylserines and phosphatic acids (PI/PS/PA)) revealed that only the PC/PE/SM fraction significantly induced resistance ( Fig. 6c–f ). Additional mass spectrometry-guided subfractionation of PC/PE/SM revealed that subfractions F3 and F6 were able to induce resistance in vivo ( Fig. 6g ). Mass spectrometry analysis of subfraction F3 derived from sCM + showed increased levels of PEs compared with F3 from sCM − . In subfraction F6 derived from sCM + , we found increased levels of lysophosphatidylcholines (LPCs) compared with F6 from sCM − ( Table 1 ). Since not all identified PEs and LPCs are commercially available for individual testing in our animal models we decided to isolate the PEs and LPCs from sCM + and test them in vivo . In parallel, we obtained purified LPC(6:0), LPC(22:0), LPC(24:0) and LPC(26:0) and mixtures of LPC and PE isolated from chicken egg and liver, respectively. Importantly, the mixtures of LPC and PE did not contain any species identified in the screen and therefore served as a control. We found that only LPCs isolated from sCM + were able to induce resistance, whereas PEs extracted from sCM + did not induce resistance in vivo ( Fig. 7a ). Both mixtures of LPC and PE lacked the ability to induce chemoresistance ( Fig. 7b ). Interestingly, the combination of saturated LPCs with cisplatin also did not induce resistance ( Fig. 7b ), suggesting that the resistance-inducing potential is restricted to the unsaturated LPCs found in sCM + . Finally, γH2AX levels in tumours treated with cisplatin in combination with LPCs isolated from sCM + were decreased similar to that observed with PIFAs. PEs isolated from sCM + also reduced γH2AX but to a lesser extent which is interesting since no effect of PE was seen on tumour volume. As expected, both the saturated LPCs and the commercial LPC mix were not able to significantly lower γH2AX levels ( Fig. 7c ). 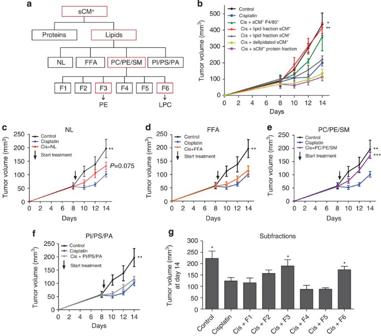Figure 6: Fractionation showed that phospholipids present in sCM+act as resistance-inducing factors. ashows schematic overview of steps used to fractionate sCM+. C26 tumour-bearing splenectomized balb/c mice were treated with either cisplatin alone or in combination with sCM+, delipidated sCM+, total lipid fraction isolated from sCM−or from sCM+or with the protein fraction isolated from sCM+. The total lipid fraction from sCM+and sCM+from F4/80+splenocytes was able to induce resistance, whereas the others did not (b). Fractionation of the total lipid fraction from sCM+by HPLC showed that only the fraction containing PC/PE/SM was able to induce resistance (c–f). Additional mass spectroscopy-guided fractionation of the PC/PE/SM fraction revealed that only subfraction F3 and F6 were able to induce chemoresistancein vivo(g). All graphs depicted show data from two independent experiments with similar outcome (n=8 per group). Statistical significance was determined by one-way analysis of variance. All compared with cisplatin alone. *P<0.05, **P<0.01. Figure 6: Fractionation showed that phospholipids present in sCM + act as resistance-inducing factors. a shows schematic overview of steps used to fractionate sCM + . C26 tumour-bearing splenectomized balb/c mice were treated with either cisplatin alone or in combination with sCM + , delipidated sCM + , total lipid fraction isolated from sCM − or from sCM + or with the protein fraction isolated from sCM + . The total lipid fraction from sCM + and sCM + from F4/80 + splenocytes was able to induce resistance, whereas the others did not ( b ). Fractionation of the total lipid fraction from sCM + by HPLC showed that only the fraction containing PC/PE/SM was able to induce resistance ( c – f ). Additional mass spectroscopy-guided fractionation of the PC/PE/SM fraction revealed that only subfraction F3 and F6 were able to induce chemoresistance in vivo ( g ). All graphs depicted show data from two independent experiments with similar outcome ( n =8 per group). Statistical significance was determined by one-way analysis of variance. All compared with cisplatin alone. * P <0.05, ** P <0.01. Full size image Table 1 Resistance-inducing factors from sCM + . 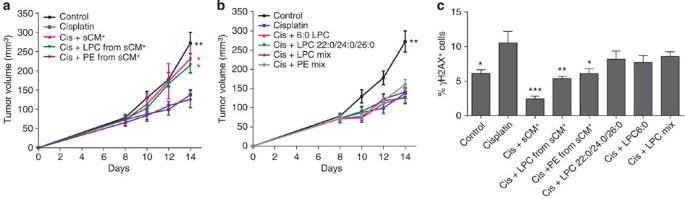Figure 7: Unsaturated LPCs secreted by splenic macrophages induce chemoresistancein vivo. LPCs isolated from sCM+induces resistance in C26 tumour-bearing mice, whereas PEs from sCM+cannot (a). To determine if the resistance-inducing potential of the identified LPCs lies in the saturated or unsaturated LPCs we tested the saturated LPCs 22:0, 24:0 and 26:0, a control short chain LPC 6:0 and commercially available LPC and PE mixtures, which does not contain any of the LPCs or PEs identified in the screen, the latter three serving as negative controls. Neither of these LPCs or LPC/PE mixes induced chemoresistance when injected together with cisplatin, indicating that resistance-inducing potential of sCM+harbours in unsaturated LPCs (b). A reduction in γH2AX was seen 4 h after co-treatment with LPCs and PEs isolated from sCM+, but not with LPC(22:0), (24;0), (26:0), (6:0) or a commercially available mix of LPC (c). All graphs depicted show data from two independent experiments (excepta, four independent experiments) with similar outcome (n=8 per group). Statistical significance was determined by one-way analysis of variance or two-tailed Studentst-test. All compared with cisplatin alone. *P<0.05, **P<0.01. Full size table Figure 7: Unsaturated LPCs secreted by splenic macrophages induce chemoresistance in vivo . LPCs isolated from sCM + induces resistance in C26 tumour-bearing mice, whereas PEs from sCM + cannot ( a ). To determine if the resistance-inducing potential of the identified LPCs lies in the saturated or unsaturated LPCs we tested the saturated LPCs 22:0, 24:0 and 26:0, a control short chain LPC 6:0 and commercially available LPC and PE mixtures, which does not contain any of the LPCs or PEs identified in the screen, the latter three serving as negative controls. Neither of these LPCs or LPC/PE mixes induced chemoresistance when injected together with cisplatin, indicating that resistance-inducing potential of sCM + harbours in unsaturated LPCs ( b ). A reduction in γH2AX was seen 4 h after co-treatment with LPCs and PEs isolated from sCM + , but not with LPC(22:0), (24;0), (26:0), (6:0) or a commercially available mix of LPC ( c ). All graphs depicted show data from two independent experiments (except a , four independent experiments) with similar outcome ( n =8 per group). Statistical significance was determined by one-way analysis of variance or two-tailed Students t -test. All compared with cisplatin alone. * P <0.05, ** P <0.01. Full size image It is becoming increasingly clear that the host plays an important role in the response to anti-cancer drugs and the development of resistance to these drugs. Here we identified a novel role for specific phospholipids released from splenic macrophages in chemotherapy resistance. Our findings show that F4/80 + /CD11b low cells residing in the spleen become activated by circulating PIFAs, and subsequently release polyunsaturated LPCs which induced systemic chemotherapy resistance via altering the DNA damage response. We show that PIFAs interfere with the early effects of DNA-damaging chemotherapeutic agents like cisplatin. In the presence of PIFAs a rapid decline in γH2AX levels was found, alleviating cell cycle arrest and restoring tumour cell proliferation to baseline levels. This was not explained by a decreased exposure to cisplatin. Since PIFAs are endogenously produced by MSCs in response to exposure to platinum analogues, and exposure to PIFAs or sCM + results in a rapid reduction of DNA damage, this could represent a physiological stress response of the body to protect itself from genotoxic agents. Our findings indicate a novel link between polyunsaturated fatty acid-signalling and the DNA damage response. Our study uncovers a number of potential drug targets to enhance chemotherapy efficacy. Here we used chemical inhibition and a genetically engineered mouse model to show that 12-S-HHT-mediated chemoresistance is dependent on BLT2 signalling. BLT2 is the low affinity receptor for leukotriene B4, however it specifically binds 12-S-HHT and initiates distinct downstream effects, different from BLT1 (ref. 13 ). Overexpression of BLT2 in breast, pancreatic and bladder tumours has been correlated to tumour progression and even to platinum resistance in ovarian cancer [15] , [16] , [17] . Our results combined with others identify BLT2 as a potential drug target to improve treatment outcome perhaps via a dual function by inhibiting the release of chemoresistance-inducing LPCs from the spleen and by inhibiting BLT2 pro-survival functions in the tumour cells itself. Alternatively, further insight into the production of the LPCs by the splenic macrophages could reveal potential drug targets that could enhance chemotherapy efficacy. Little is known about LPCs in cancer and chemotherapy resistance and no receptors have yet been described. It remains to be determined whether these specific LPCs act through specific receptors or directly. Taken together our results have uncovered a systemic signalling network of PIFAs and LPCs generated by MSCs and splenic cells that render tumour cells resistant to chemotherapy via alterations in the DNA damage response of tumour cells. Reagents 12-S-HHT, U-75302 and LY255283 were purchased from Cayman Chemicals. 16:4(n−3) was a kind gift from Dr Ishihara [18] . The following antibodies were used for magnetic bead sorting: rat anti-mouse F4/80, rat anti-mouse CD169 (both from AbD serotec), anti-human and mouse CD11b-FITC, anti-mouse CD11c microbeads, anti-mouse CD49b (DX5) microbeads, (all from Miltenyi biotec), rat anti-mouse CD45R (B220), rat anti-mouse CD3-FITC (both from ebioscience), anti-rat IgG microbeads and anti-FITC microbeads (both from Miltenyi biotec). For FACS analysis the following antibodies were used: rat anti-mouse F4/80-FITC and rat anti-mouse CD11b-APC (both from ebioscience). For immunohistochemical staining the following antibodies were used: anti-γH2AX (Cell Signaling Inc), anti-BrdU (Abcam), anti-pH3 (Upstate/Millipore Corporation), Powervision-HRP Goat-anti-Rabbit (Novocastra/Leica Microsystems) and Goat-anti-Rabbit Alexa-568 (Life Technologies). Animal models C26 and LLC cells were implanted in balb/c and C57bl/6 (both from Charles River) mice, respectively. For all experiments 8–10-week-old male mice were used. At day 0 the mice were injected subcutaneously with 1 × 10 6 (for C26) or 0.5 × 10 6 (for LLC) tumour cells. Mice were splenectomized 1 day after tumour cell injection. At day 8 (C26) or day 10 (LLC) when the tumours were at a palpable size of 50–100 mm3, animals were randomized into groups and treatment was started. The mice received an intraperitoneal injection of cisplatin 6 mg kg −1 and blinded tumour volume measurements were done once every 2 days using a caliper. Tumour volume was determined as length × width 2 × 0.5. Control mice received the appropriate vehicles. Concomitantly with the chemotherapy treatment, some mice received subcutaneous injection of conditioned medium from splenocytes cultured in the presence (sCM + ) or absence (sCM − ) of PIFAs. Generation of the BLT2 −/− mice is described in the study by Mathis et al. [13] Therapy was started when tumours reached 50–100 mm 3 and tumour growth was monitored as described above. Endpoints were determined as a tumour volume of >1000, mm 3 . All experimental animal procedures conducted in Utrecht (the Netherlands) were approved by the University Medical Center Animal Ethics Committee and were in agreement with the current Dutch Laws on animal experiments. All experimental animal procedures conducted in Louisville (KY, USA) were approved by the University of Louisville Animal Care and Use Committee. To show a difference of 20% in tumour volume with a s.d. of 10% and a type I error ( α ) of 5% using a power of 90% a minimal of eight mice per treatment group are required. Cell lines C26 and LLC cells (both from ATCC) were grown in DMEM (4,5 gr/l glucose)+5% FCS at 5% CO2 and 37 °C. Murine MSCs were grown in DMEM (1 gr/l glucose)+20% FCS at 5% CO2 and 37 °C. Liver metastasis model C26 tumour cells (5*10 4 cells) were injected intra-splenically in balb/c mice and allowed to migrate to the liver. One day after tumour cell injection the spleens were removed to prevent local tumour growth. Six days after tumour cell injection the mice were either left untreated, treated with cisplatin or with cisplatin and CM+ from the MSCs. After 4 days the livers were harvested, weighted and the hepatic replacement area was determined. Production of sCM from splenocytes Spleens from splenectomized mice were used to make sCM. Single cell suspensions were made from the spleens and red blood cells (RBCs) were lysed using RBC lysis buffer (155 mM NH 4 Cl, 10 mM KHCO 3 and 0.1 mM EDTA). Splenocytes were incubated in serum-free medium (DMEM 4,5 g glucose per l) with 20 nM 12-S-HHT and/or 25 nM 16:4(n−3) for 1 h at 5% CO2 and 37 °C. After incubation the supernatant from the splenocytes was harvested, filtered through a 0.2 μM filter and stored at −80 °C until use. Magnetic-activated cell sorting of splenic cell populations The spleens were processed into the same way as described for the production of sCM. After RBC lysis the splenocytes were resuspended in FACS buffer (1% BSA, 5 mM EDTA in PBS pH 7.4) and counted. Next, the cells were incubated with primary antibodies rat anti-mouse F4/80, rat anti-mouse CD11b-FITC, rat anti-mouse CD169, anti-mouse CD11c microbeads, anti-mouse CD49b (DX5) microbeads, rat anti-mouse CD45R (B220), rat anti-mouse CD3-FITC at a concentration of 3 μl per 1 × 10 7 cells in 100 μl for 30 min on ice. After incubation, the cells were washed in FACS buffer and incubated with secondary antibodies (goat anti-rat microbeads or goat anti-FITC microbeads) at a concentration of 5 μl per 1 × 10 7 cells in 100 μl for 15 min on ice. Again the cells were washed after antibody incubation and resuspended in FACS buffer and separated according to the manufacturer’s instructions using LS columns (Miltenyi Biotec). Labelled cells were spun and incubated in SFM with 20 nM 12-S-HHT and/or 25 nM 16:4(n−3) for 1 h at 5% CO2 and 37 °C. The supernatant was harvested and stored as described in the section ‘Production of sCM from splenocytes’. For the BLT1 and BLT2 inhibitor experiments, the isolated macrophages were incubated with LY255283 (800 nM) or U-75302 (500 nM) for 1 h prior to addition of HHT (20 nM) or 16:4(n−3) (25 nM). Liposomal clodronate administration All tumour-bearing mice received 200 μl of liposomal clodronate suspension (containing 2 mg clodronate) via intravenous injection 2 and 4 days prior to chemotherapy treatment to ensure maximal depletion of splenic macrophages at the time of treatment. At day 8 (for balb/c mice) or day 10 (for C57Bl/6 mice) the mice were either left untreated, treated with cisplatin (6 mg kg −1 ) alone or in combination with PIFAs (20 nM HHT and 25 nM 16:4(n−3) or sCM + from F4/80 + spleen macrophages. FACS analysis of liposomal clodronate-treated mice To determine maximal depletion of spleen macrophages FACS profiles were made from non-tumour-bearing mice 2, 4 or 8 days after a single liposomal clodronate injection. In brief, single cell suspensions made from the spleen and RBCs were lysed as described in the section ‘Production of sCM from splenocytes’. Next, the splenocytes were incubated with F4/80-FITC and CD11b-APC (concentration 1 μl per 1 × 10 7 cells per 100 μl) or corresponding isotype controls (FITC and APC both from ebiosciences) in FACS buffer for 30 min on ice. Samples were analyzed using a FACSCalibur from BD biosciences. FACS sorting splenic populations Spleens were prepared as described in the section ‘FACS analysis of liposomal clodronate-treated mice’ and the F4/80 + /CD11b low , F4/80 + /CD11b high , F4/80 − /CD11b high and F4/80 − /CD11b − populations were sorted using a FACSAria III from BD biosciences. Gates for sorting were set according to unstained and isotype control-stained samples. Quantitative PCR analysis of BLT2 RNA was extracted from FACS-sorted splenic population, C26 and LLC cells using TriZol (invitrogen). complementary DNA was synthesized using Superscript II (invitrogen) according to manufacturer’s protocol. Primers used for detection of BLT2: forward: 5′-ACCATGGAACTCCGAACTAC-3′, reverse: 5′-ACTGTCTTTCTCCGTCTTGC-3′. As a control GADPH was used; forward: 5′-ATGCAGGGATGATGTTCT-3′. reverse: 5′-GTCATCCATGACAACTTT-3′. Immunohistochemistry and immunofluorescence For immunohistochemistry experiments, tumours were harvested 0.5, 1, 2, 4 and 12 h after therapy. Formaldehyde-fixed paraffin-embedded tumour sections were deparaffinated and rehydrated in a series of xylene and alcohol, incubated in a buffer containing 5% H2O2 to block endogenous peroxidase, and antigen retrieval was performed by cooking slides in citrate buffer. Tissues were blocked with goat serum (Life Technologies Europe BV) and incubated with primary antibodies: 1:200 anti-γH2AX (Cell Signalling Inc., #2577, USA) or 1:200 anti-BrdU (Abcam, #ab6326, Cambridge, UK) overnight at 4 °C. Powervision-HRP Goat-anti-Rabbit (1:2000; Novocastra/Leica Microsystems, Germany) was used as secondary antibody, followed by DAB/H2O2 and counterstaining with haematoxyline. For immunofluorescent stainings, anti-pH3 (#06-570, Upstate/Millipore Corporation, USA) was used 1:250 overnight at 4 °C, followed by the secondary antibody 1:500 Goat-anti-Rabbit Alexa-568 (#A11036, Life Technologies) and DAPI staining (#33342, Hoechst/Life Technologies). Analysis was performed using a grid with 36 intersection points. At least 10 fields per tumour were analyzed. Measuring platinum concentrations Mice were treated with cisplatin (6 mg kg −1 ) with or without co-administration of PIFAs. Thirty minutes after therapy, tumours were harvested, weighed and snap frozen. Either DNA was isolated or nuclear/cytosolic extractions were performed, followed by measuring platinum concentration as previously described [19] , [20] , [21] . In brief, for DNA isolation tumours were homogenized using Douncer homogenizers in Tris-HCl buffer, followed by addition of NH 4 HCO 3 , SDS and Proteinase K, overnight digestion at 42 °C and protein precipitation by adding saturated 6 M NaCl, vigorous shaking and spinning. The DNA was precipitated from the supernatant by addition of pure EtOH, washed twice in 75% EtOH, airdried and dissolved in dH2O. For nuclear and cytoplasmic extraction, snap frozen tumour tissues were homogenized in hypotonic lysis buffer with addition of NP-40 and protease/phosphatase inhibitors, which will lyse the cytoplasmic fraction. Subsequently, the nuclei were lysed with ice-cold nuclear extraction buffer with protease/phosphatase inhibitors. Protein content was measured using a spectophotometer and control western blots were performed. DNA, nuclear and cytoplasmic fractions were hydrolyzed and analyzed by inductively coupled plasma mass spectrometry [22] , [23] , [24] . Lipid fractionation and mass spectrometry analysis of sCM + Total lipids from culture media of sCM were extracted using a modified Bligh & Dyer extraction according to the study by Retra et al. [24] Total lipid fraction was separated into four fractions (neutral lipids), free fatty acids, two phospholipid fractions (PC/PE/SM and PI/PS/SM) by solid phase extraction according to the study by Kim et al. [22] The PC/PE/SM fraction was further fractionated into separate lipid classes by hydrophilic interaction liquid chromatography as described by the study by Brouwers et al. [23] The HPLC output was split into two flows (1:10 ratio), of which one was lead to a mass spectrometer to monitor the separation process, the other major flow was used to collect lipid classes. LPC analysis was performed using a modified method by Retra et al. [24] Here the HPLC column was replaced by a fused core HALO C18 column (Biotech, Onsala, Sweden). To increase sensitivity, LPCs were detected in multiple reaction monitoring mode, in which a collection of 36 different LPC masses (14:0 to 26:6 LPC) were monitored and confirmed by the formation of a phosphocholine fragment of 184 m/z (collision energy was 55 V). Furthermore, the fatty acid composition of the LPCs was confirmed by the presence of the corresponding fatty acid fragment in a second mass spectrometry analysis. Resulting fractions were speed-vacuum dried and dissolved in ethanol and diluted into PBS before injection in mice. Statistical analysis All data are presented [18] as mean±s.e.m.. Statistical significance for all animal experiments in which tumour volumes were assessed was determined by one-way analysis of variance with Tukey correction for multiple testing. A value of P <0.05 was considered to be statistically significant. All other data was analyzed using a two-tailed Students t -test. A P -value<0.05 was considered statistically significant. A Levene’s test was used to determine if variance between groups was comparable. Animals were excluded from analysis if two or more tumour measurements were significant outliners compared with the rest using the Grubbs outlier test ( α =0.05). How to cite this article: Houthuijzen, J. M. et al. Lysophospholipids secreted by splenic macrophages induce chemotherapy resistance via interference with the DNA damage response. Nat. Commun. 5:5275 doi: 10.1038/ncomms6275 (2014).